High-sensitivity accelerometer composed of ultra-long vertically aligned barium titanate nanowire arrays A configuration that shows great promise in sensing applications is vertically aligned piezoelectric nanowire arrays that allow facile interfacing with electrical interconnects. Nano-electromechanical systems developed using piezoelectric nanowires have gained interest primarily for their potential in energy harvesting applications, because they are able to convert several different sources of mechanical energy into useful electrical power. To date, no results have demonstrated the capability to use aligned piezoelectric nanowire arrays as a highly accurate nano-electromechanical system based dynamic sensor with a wide operating bandwidth and unity coherence. Here we report the growth of vertically aligned (~45 μm long) barium titanate nanowire arrays, realized through a two-step hydrothermal synthesis approach, and demonstrate their use as an accurate accelerometer. High sensitivity of up to 50 mV g −1 is observed from the sensor composed of vertically aligned barium titanate nanowire arrays, thus providing performance comparable to many of the commercial accelerometer systems. Piezoelectric materials offer coupling between mechanical and electrical energy, allowing them to be effectively fabricated as transducers that can be configured as either sensors or actuators. Many sensing applications incorporate piezoelectric materials, because they require minimal signal conditioning and have wide bandwidth well into the MHz range. Furthermore, piezoelectric materials have been found particularly well suited for micro-electromechanical systems (MEMS), as the energy density does not decrease with the dimensions, as is the case in electromechanical or magneto-mechanical systems. When applied in MEMS applications, piezoceramics are typically constrained to a thin film, which places certain limits on the design of the device and typically requires the use of the lower k 31 piezoelectric coefficient [1] . An alternative configuration that shows great promise as a sensor is vertically aligned piezoelectric nanowire (NW) arrays that allow for facile interfacing with electrical interconnects. The NW form of these materials offers considerable advantages due to the high aspect ratio, which leads to highly deformable structures [2] , [3] and size effects [4] that act to enhance the piezoelectricity of the ceramic. Consequently, piezoelectric NWs have tremendous potential to be applied in the emerging field of nano-electromechanical systems (NEMS). NEMS developed using piezoelectric NWs have received attention primarily for their potential in power harvesting applications, because they are able to convert several different sources of mechanical energy such as sound waves [5] , ultrasonic waves [6] , [7] , [8] , vibrational energy [9] , [10] , atomic force microscope tip-induced stimulus [11] , [12] and biomechanical energy [13] , [14] into useful electric power. The direct piezoelectric effect responsible for the energy harvesting behaviour is identical to the response required for sensing. However, energy harvesting represents a more simplistic operation, as the voltage output can contain significant noise, requires little to no correlation to the input energy and places no limits on the bandwidth or stability of the response. On the contrary, a functional sensor must produce an output that can be very accurately correlated to the force (mechanical measurands) acting on it and without noise that would limit the sensitivity and measurement floor. In recent years, ZnO NWs have garnered significant interest for sensing and energy harvesting; however, ZnO possess both a low piezoelectric coupling coefficient and semiconductor behaviour unlike many ferroelectric ceramics and, therefore, can result in sensors with low sensitivity and a high noise floor [15] . Although ZnO NWs have a low dielectric constant, which increases its voltage output, the performance has been very limited and no sensor has been demonstrated to produce a high coherence between the input and output across the sensor’s bandwidth [5] , [16] , [17] , [18] . To improve the electromechanical coupling performance of the NW-based devices, ferroelectric perovskite nanostructures such as PZT (PbZr x Ti 1-x O 3 ) (refs 19 , 20 , 21 ) NWs have been explored; however, they have only been applied for energy harvesting applications. Moreover, environmental concerns over the use of lead-based piezoelectric materials have motivated the need to develop and utilize lead-free piezoelectric nanostructures for sensors [22] . Among the lead-free ceramics, barium titanate (BaTiO 3 ) is the most studied and possesses one of the highest coupling values. However, before this study, no synthesis method for the growth of vertically aligned BaTiO 3 NW arrays had been demonstrated, and thus this high-performance lead-free material has received little attention in the NW form. Here we describe the synthesis of ultra-long (up to 45 μm), vertically aligned BaTiO 3 NW arrays that is achieved through a low-cost, two-step hydrothermal growth approach. We show that not only are these NWs piezoelectric and could function as energy harvesting material, but that the NW arrays can be used to fabricate a NEMS accelerometer with high sensitivity, unity coherence and wide operating bandwidth. High sensitivity of ~50 mV g −1 is demonstrated from the NEMS sensor composed of vertically aligned BaTiO 3 NW arrays, thus providing performance comparable to many of the commercial accelerometer systems. In addition, the sensitivity of the BaTiO 3 NW sensor (~50 mV g −1 ) is observed to be much higher than the sensitivity of ZnO NW sensor (~2.5 mV g −1 ) when direct comparison is performed under the same testing conditions, thereby validating the superior sensing performance of the ultra-long, vertically aligned BaTiO 3 NW arrays. Synthesis and characterization of BaTiO 3 NW arrays A hydrothermal process is employed to grow vertically aligned BaTiO 3 NW arrays that is of low cost and is scalable, allowing batch processing and control over the length and diameter of the NWs. An important feature of this synthesis procedure is that the surfaces can be tailored using MEMS processing. For example, isolated patches of NWs can be fabricated such that sensing arrays can be used to achieve extremely high spatial resolution. The BaTiO 3 NW arrays are realized through the conversion of vertically aligned sodium titanate NW arrays grown on an oxidized titanium substrate. The nanowires’ microstructure was characterized using scanning electron microscopy (SEM), as shown in Fig. 1a , and high-resolution transmission electron microscope (HRTEM). The BaTiO 3 NW arrays span a length of 45 μm and the diameter of the individual NWs are ~600 nm. These dimensions were chosen such that the NWs are sufficiently rigid to allow their use in compression without buckling or wicking together during drying [23] . The crystallographic structure of the NWs was analysed using X-ray diffraction (XRD), and the XRD pattern in Fig. 1b shows the NWs are BaTiO 3 (JCPDS number 5-0626; see Supplementary Figure S1 for XRD pattern of all materials used in BaTiO 3 NW synthesis). The HRTEM image of the as-prepared sodium titanate NW precursors showed a single crystalline structure as shown in Fig. 1c and transforms into a single crystalline BaTiO 3 NW after a second hydrothermal reaction containing barium ions as shown in Fig. 1d . To retain the vertically aligned morphology of the precursor sodium titanate NW arrays, the concentration of the barium (Ba 2+ ) ions used in the hydrothermal treatment is held to a minimum. This structural transformation from sodium titanate NW precursor to a single-crystal BaTiO 3 NW results due to the diffusion of the barium (Ba 2+ ) ions into the sodium titanate NWs from the temperature-assisted hydrothermal ion-exchange reaction [24] , [25] . 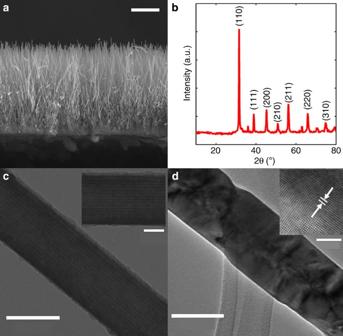Figure 1: Characterization of BaTiO3NW arrays. (a) A cross-sectional SEM image of BaTiO3NW arrays (scale bar, 20 μm). (b) XRD spectrum from the BaTiO3NW arrays (JCPDS number 5-0626) synthesized using sodium titanate NW arrays as precursor. (c) An HRTEM image of the single-crystal sodium titanate NW precursor (scale bar, 100 nm) with the inset showing the clear crystal lattice fringes (scale bar, 25 nm). (d) An HRTEM image of the single BaTiO3NW showing single-crystal structure after ion transfer (scale bar, 100 nm), with the inset showing the clear crystal lattice fringes (scale bar, 5 nm; arrows are used to indicate the crystal lattice spacing distance of 4.12 Å). Figure 1: Characterization of BaTiO 3 NW arrays. ( a ) A cross-sectional SEM image of BaTiO 3 NW arrays (scale bar, 20 μm). ( b ) XRD spectrum from the BaTiO 3 NW arrays (JCPDS number 5-0626) synthesized using sodium titanate NW arrays as precursor. ( c ) An HRTEM image of the single-crystal sodium titanate NW precursor (scale bar, 100 nm) with the inset showing the clear crystal lattice fringes (scale bar, 25 nm). ( d ) An HRTEM image of the single BaTiO 3 NW showing single-crystal structure after ion transfer (scale bar, 100 nm), with the inset showing the clear crystal lattice fringes (scale bar, 5 nm; arrows are used to indicate the crystal lattice spacing distance of 4.12 Å). Full size image NW NEMS sensor configuration The sensor was fabricated from the vertically aligned BaTiO 3 NW arrays by first removing the NW arrays from the oxidized titanium substrate on which they were grown to a borosilicate glass substrate. The NW arrays can be readily handled after release from the oxidized growth substrate by immersing in dilute HCl solution. The NW arrays were then bonded to the glass substrate using silver epoxy, which acted as a bottom electrode, and a thin solder foil (Sn60Pb40) was applied to the top surface of the NWs, which acted as the top electrode (see Supplementary Fig. S2a,b for images on handling of NW arrays and the fabrication process flow). The NW arrays with the solder foil were then heated to 150 °C for 1 h to improve bonding with the NWs (see Supplementary Fig. S3a–c for the NW adhesion between the two electrodes following the heating in the fabrication process). The two electrodes sandwiched the vertically aligned BaTiO 3 NW arrays, with the glass acting as the substrate for handling and mounting to the excitation source as shown in the schematic in Fig. 2a (see Supplementary Fig. S4a for an image of the fabricated BaTiO 3 NW acceleration sensing device and Supplementary Fig. S3a,b for the cross-sectional SEM images of the BaTiO 3 NWs between the two electrodes). After fabrication, the BaTiO 3 NW arrays were polled by applying a DC field of ~75 kV cm −1 across the two electrodes of the sensor for 12 h. The denser layer of BaTiO 3 NWs near the base electrode assists to insulate the sandwich structure from breakdown during the poling process [26] , [27] . High-voltage poling is performed to ensure the dipoles in the BaTiO 3 NW arrays align in the electric field direction, which is normal to the plane of the two electrodes and along the orientation of the NWs. Poling is not required for non-ferroelectric piezoceramic materials such as ZnO; however, it is critical for the piezoelectric function of the single-crystal BaTiO 3 NWs developed here. 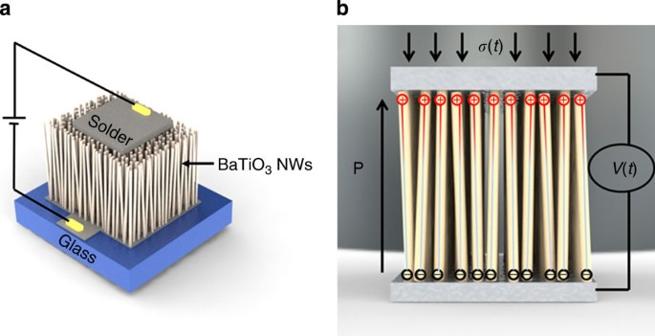Figure 2: Sensor device configuration. (a) Schematic diagram of sensor device using BaTiO3NW arrays. (b) Schematic of piezoelectric voltage generation from NWs. Polarization direction (P) represents the alignment direction of the dipoles. Application of dynamic stress (σ(t)) on NW arrays produces voltage (V(t)) generation. Figure 2: Sensor device configuration. ( a ) Schematic diagram of sensor device using BaTiO 3 NW arrays. ( b ) Schematic of piezoelectric voltage generation from NWs. Polarization direction ( P ) represents the alignment direction of the dipoles. Application of dynamic stress ( σ(t) ) on NW arrays produces voltage ( V(t) ) generation. Full size image For the fabricated sensor, acceleration is determined by mounting the sensor to a vibrating surface and then measuring the piezoelectric potential formed due to the dynamic stress resulting from the inertia of the solder on the NWs’ top surface ( Fig. 2b ). If the stress applied is constant or removed from the NWs, the accumulated charge is dissipated and the resulting piezoelectric voltage would diminish, which correlates well with the piezoelectric material’s limitation to dynamic sensing applications. The piezoelectric voltage developed depends on the direction, amplitude and frequency of the stress that is applied on the sensor, as it follows the dynamic characteristics of a linear system. Here the sensor’s base is fixed to a permanent magnet shaker that acts as the acceleration source so that the inertia from the top electrode supplies the necessary time varying compressive and tensile stress on the vertically aligned BaTiO 3 NW arrays. The stress on the NWs is proportional to the acceleration of the base and, thus, the NWs produce a voltage proportional to the acceleration of the device. The open-circuit piezoelectric voltage output is measured using a high impedance voltage follower (1 TΩ), and all measurements are performed inside a grounded faraday cage to eliminate the effects of extraneous noise on the sensor output voltage (see Supplementary Fig. S4b,c for images of the experimental test setup). In addition, the voltage follower (LTC6240CS8) used has a very low-input bias current (0.2 pA) to function efficiently as a voltage measuring interface circuit for the piezoelectric NW sensor (see Supplementary Fig. S5 for schematic of the circuit representation). The BaTiO 3 NW sensor was mounted on the base of the shaker that acts as the acceleration source beside a reference accelerometer that measures the true acceleration. The voltage follower is placed in near proximity to the sensor, such that leakage current is minimized during measurement from the sensor source, which has high input impedance (low capacitance), and also to counteract the effects of parasitic capacitance that could adversely affect the sensor’s actual sensitivity (see Supplementary Fig. S4c ). The grounded faraday cage acting as a noise shield from electromagnetic interference helps to improve the signal-to-noise ratio of the sensor; therefore, there is little presence of detrimental extrinsic noise at the input and output points to affect the sensor’s linear characteristics (see Supplementary Fig. S6a for voltage noise floor power measured from the experimental setup). Frequency response characterization of NEMS sensor The dynamic characteristics of the novel compression-type BaTiO 3 NW-based accelerometer are described using the frequency response function (FRF). The FRF defines the relative magnitude and phase between the reference sensor (PCB 352C22), which produces an accurate measure of the input acceleration acting on the device, and the output piezoelectric voltage of the NW sensor. In past efforts to characterize piezoelectric NW-based sensors [5] , [16] , [17] , [18] , the linearity, bandwidth and coherence of the devices were never investigated. It is critical that these characteristics be considered, as they, along with the sensitivity, define the ultimate performance of the sensor. The linearity and validity of the sensor’s measurement are evaluated using the coherence function, which represents the degree of linearity between the input base acceleration (instrumentation-grade accelerometer) and the output piezoelectric voltage of the NW sensor [28] . The coherence is a non-linear function with values from 0 to 1, with 1 defining a perfect linear relationship between the two signals and, therefore, an accurate measure of the input [29] . The coherence drops below unity in the presence of noise, non-linearity in the measured oscillations or spurious frequencies in the output. A stationary Gaussian white noise signal is used for excitation of the base, due to its spectral density being flat across the entire test frequency that spans up to 10 kHz (see Supplementary Fig. S6b for input acceleration spectral density). The thin film of solder that was attached to the top of the NWs as a top electrode provides the proof mass (16 mg) for acceleration sensing and is utilized in two different settings to analyse the sensing behaviour of the BaTiO 3 NWs (see Supplementary Table S1 for the properties of the fabricated sensor). The solder is heated to form a stable rigid contact with the NWs, resulting in a flat band magnitude response in FRF ( Fig. 3a ) of up to 10 kHz with only a slight phase variation ( Fig. 3b ). This flat band region is essential for characterizing the sensor’s operating frequency range and is observed due to the resonant frequency of the sensor device falling above the bandwidth of the electromagnetic shaker used for excitation. The coherence function is very strong, reaching unity across the entire test frequency range, and thereby demonstrates the accurate measurement of acceleration from the NW arrays ( Fig. 3c ). A mean sensitivity of ~800 μV g −1 is obtained in the ±3 dB flat band region in the FRF magnitude that spans across the entire frequency range where ‘g’ represents the acceleration due to gravity. Here the sensitivity is lower but the operating bandwidth of the sensor spans up to 10 kHz. 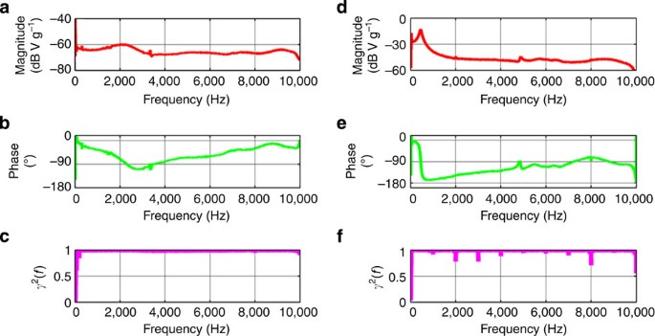Figure 3: Dynamic response characterization of BaTiO3NW sensor. (a) FRF illustrated by magnitude in dB scale of V g−1, (b) phase angle in degree and (c) the coherence function (γ2(f)) of BaTiO3NW sensor with a heated solder as the top electrode demonstrated flat band region with strong unity coherence up to 10,000 Hz from white noise excitation. (d) FRF illustrated by magnitude in dB scale of V g−1, (e) phase angle in degree, and (f) the coherence function (γ2(f)) of BaTiO3NW sensor with an added mass on the top electrode produced a resonance frequency at 450 Hz associated with 90° phase shift and demonstrated an enhanced sensitivity (~50 mV g−1) in the ±3 dB flat band region of up to 300 Hz. Figure 3: Dynamic response characterization of BaTiO 3 NW sensor. ( a ) FRF illustrated by magnitude in dB scale of V g −1 , ( b ) phase angle in degree and ( c ) the coherence function ( γ 2 (f) ) of BaTiO 3 NW sensor with a heated solder as the top electrode demonstrated flat band region with strong unity coherence up to 10,000 Hz from white noise excitation. ( d ) FRF illustrated by magnitude in dB scale of V g −1 , ( e ) phase angle in degree, and ( f ) the coherence function ( γ 2 (f) ) of BaTiO 3 NW sensor with an added mass on the top electrode produced a resonance frequency at 450 Hz associated with 90° phase shift and demonstrated an enhanced sensitivity (~50 mV g −1 ) in the ±3 dB flat band region of up to 300 Hz. Full size image On addition of mass to the top electrode, the resonant frequency can be brought down to a frequency measureable within the electromagnetic shaker’s bandwidth, which confirms the existence of a high-frequency resonance of the unloaded device. By considering the NW arrays to act as a spring, the increased mass will decrease the resonant frequency (450 Hz) as observed in the FRF magnitude in Fig. 3d associated with 90° FRF phase shift at the resonant frequency ( Fig. 3e ). The added mass on the sensor’s top electrode enhances the dynamic stress level on the sensing NWs, resulting in improved piezoelectric voltage generation from the sensor. The FRF from the loaded sensor substantiates this behaviour, as there is a considerable increase in the magnitude, which equates to a higher mean sensitivity of ~50 mV g −1 in the ±3 dB bandwidth of the sensor that spans up to 300 Hz. The coherence is still observed to be unity, confirming the accuracy of the FRF measurement made from the loaded sensor ( Fig. 3f ). Here the sensitivity is higher but the operating bandwidth is reduced, contributing to a trade-off in the performance of the sensor. A sine wave excitation is performed to confirm frequency preservation observed from the coherence function. From input sinusoidal acceleration amplitude of 1 g, root mean square (RMS) sensitivity is calculated and shows a peak of ~180 mV g −1 at the resonance frequency (450 Hz) of the loaded sensor as shown in Fig. 4a . A high mean RMS sensitivity of ~50 mV g −1 is obtained up to 300 Hz, which correlates well with the FRF magnitude, justifying that the loaded sensor is well suited for accurate low-frequency acceleration measurements. Moreover, the acceleration noise floor (minimum detectable signal) from the NW accelerometer is considerably lower (~0.005 g) owing to the higher sensitivity and lower-voltage noise floor (RMS ~250 μV) in the operating bandwidth. Peak-to-peak voltage ( V pp ) of ~80, ~85 and ~130 mV is obtained from 100 ( Fig. 4b ), 200 ( Fig. 4d ) and 300 Hz ( Fig. 4f ), respectively, for a 1-g input acceleration sinusoidal amplitude with the corresponding detailed shapes shown in Fig. 4c,e,g . Higher V pp of ~340 mV is obtained from only 1 g acceleration amplitude from the sensor near resonance ( Fig. 4h,i ; see Supplementary Fig. S7a,b for detailed shape of acceleration and voltage that is in phase at 100 Hz and 90° out of phase near resonance at 450 Hz). Therefore, the results recorded from the novel BaTiO 3 NW accelerometer demonstrate the potential of the NWs to have a dual role in sensing and in power-harvesting applications. 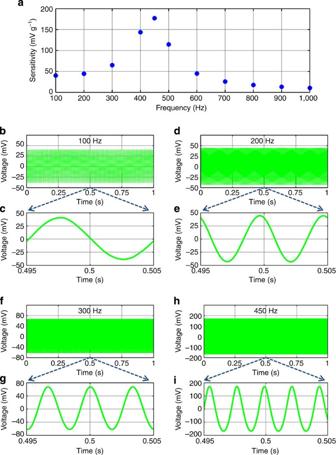Figure 4: Sinusoidal excitation on BaTiO3NW sensor. (a) RMS sensitivity from frequencies of 100–1,000 Hz. (b) Voltage measured at 100 Hz with (c) showing the detailed shape. (d) Voltage measured at 200 Hz with (e) showing the detailed shape. (f) Voltage measured at 300 Hz with (g) showing the detailed shape. Voltage measured at 100 (b), 200 (d) and 300 Hz (f) from 1 g amplitude acceleration input correlates well with the mean RMS sensitivity of ~50 mV up to 300 Hz. (h) Voltage measured near resonant frequency (450 Hz) with (i) clearly showing the detailed shape of a highVppof 342 mV produced at resonance from 1 g amplitude acceleration input. Figure 4: Sinusoidal excitation on BaTiO 3 NW sensor. ( a ) RMS sensitivity from frequencies of 100–1,000 Hz. ( b ) Voltage measured at 100 Hz with ( c ) showing the detailed shape. ( d ) Voltage measured at 200 Hz with ( e ) showing the detailed shape. ( f ) Voltage measured at 300 Hz with ( g ) showing the detailed shape. Voltage measured at 100 ( b ), 200 ( d ) and 300 Hz ( f ) from 1 g amplitude acceleration input correlates well with the mean RMS sensitivity of ~50 mV up to 300 Hz. ( h ) Voltage measured near resonant frequency (450 Hz) with ( i ) clearly showing the detailed shape of a high V pp of 342 mV produced at resonance from 1 g amplitude acceleration input. Full size image Validation of piezoelectricity from BaTiO 3 NW sensor A verification of the piezoelectric behaviour from the BaTiO 3 NW accelerometer was performed by heating it above the Curie temperature of the BaTiO 3 at 120 °C to relax the orientation of the electric dipoles, which would eliminate the formation of a net charge on the sensor under stress [30] . The depoled NW sensor was then tested under white noise excitation and demonstrated to produce no measureable signal in FRF with loss in coherence, which confirms the transition from tetragonal phase to cubic phase of the BaTiO 3 NWs on heating above the Curie temperature ( Fig. 5a–c ) [29] . In addition, poling/depoling/re-poling analysis and switching polarity test were performed for BaTiO 3 NEMS sensor to validate piezoelectricity from ferroelectric BaTiO 3 NW arrays (see Supplementary Figs S8 and S9 ) [31] , [32] . To further substantially confirm piezoelectricity, the poling voltage (DC field 75 kV cm −1 ) was reversed in polarity to switch the polarization direction ( P ) of the electric dipoles within the ferroelectric BaTiO 3 NW arrays of the same sensor. This switching of polarization direction ( P ) in two opposite directions was performed to witness a reversal in the peaks (polarity) of the output voltage response ( V ) from the same NW sensor for the same mechanical deformation when connected with same terminals to the voltage follower as shown in Fig. 5d–f . This result demonstrates the switchable polarization direction ( P ) property of ferroelectric BaTiO 3 NW arrays and its influence on output voltage response ( V ) to conclusively validate piezoelectricity [33] . These results thereby confirm the presence of piezoelectric property in the ferroelectric BaTiO 3 NW arrays that was responsible for showing high sensitivity, unity coherence and excellent linearity in a wide operating bandwidth from the NW accelerometer that was poled before testing. 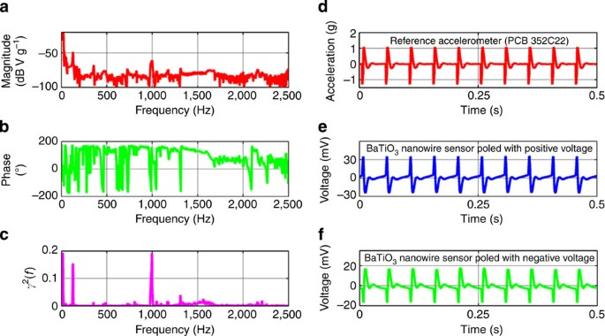Figure 5: Influence of depoling and switchable polarization direction. (a) FRF illustrated by magnitude in dB scale of V g−1, (b) phase angle in degree and (c) the coherence function (γ2(f)) of BaTiO3NW sensor under white noise excitation when heated to 150 °C for 3 h (Curie temperature,TC=120 °C) shows the loss in piezoelectric behaviour from depoling as the electric dipoles in the NWs have been relaxed from their oriented poled state to random directions. (d) Acceleration measured by reference accelerometer (PCB 352C22) to low-frequency pulse input. (e) The output voltage response (V) from the same BaTiO3NW sensor to pulse input is measured after poling it with positive voltage (75 kV cm−1DC field) and (f) then poling it with negative voltage (−75 kV cm−1DC field) to investigate the influence of reversing the polarization direction (P) on the output. The sensor is connected with same terminals to voltage follower to demonstrate the reversing output voltage signal (V) (e,f) from the same mechanical deformation by switching the polarization direction (P) to confirm that the measured voltage response from the sensor is generated by ferroelectric BaTiO3NW arrays. Figure 5: Influence of depoling and switchable polarization direction. ( a ) FRF illustrated by magnitude in dB scale of V g −1 , ( b ) phase angle in degree and ( c ) the coherence function ( γ 2 (f) ) of BaTiO 3 NW sensor under white noise excitation when heated to 150 °C for 3 h (Curie temperature, T C =120 °C) shows the loss in piezoelectric behaviour from depoling as the electric dipoles in the NWs have been relaxed from their oriented poled state to random directions. ( d ) Acceleration measured by reference accelerometer (PCB 352C22) to low-frequency pulse input. ( e ) The output voltage response ( V ) from the same BaTiO 3 NW sensor to pulse input is measured after poling it with positive voltage (75 kV cm −1 DC field) and ( f ) then poling it with negative voltage (−75 kV cm −1 DC field) to investigate the influence of reversing the polarization direction ( P ) on the output. The sensor is connected with same terminals to voltage follower to demonstrate the reversing output voltage signal ( V ) ( e , f ) from the same mechanical deformation by switching the polarization direction ( P ) to confirm that the measured voltage response from the sensor is generated by ferroelectric BaTiO 3 NW arrays. Full size image Comparison with ZnO NW NEMS sensor To demonstrate the superior sensing performance of the ultra-long, vertically aligned BaTiO 3 NW arrays over conventional ZnO NW arrays, a direct comparison was made with a ZnO NW-based sensor that was characterized through the same testing procedure. The ZnO NW sensor was fabricated from ZnO NW arrays grown on Au/Si substrate, using seedless hydrothermal synthesis procedure [34] , [35] . The ZnO sensor has the same electrode configuration with a thin solder foil as the top electrode but with the Au layer on a Si substrate as the bottom electrode sandwiching the ZnO NW arrays (see Methods section for the details on the synthesis of ZnO NW arrays and fabrication of the ZnO sensor and Supplementary Fig. S10a for the cross-sectional SEM image of the ZnO NW arrays). The loaded ZnO sensor with the same proof mass as the loaded BaTiO 3 sensor was then excited with white Gaussian noise to characterize the FRF (see Supplementary Table S2 for the properties of ZnO sensor). A resonant magnitude peak at 500 Hz associated with the 90° phase shift was detected on the FRF of the loaded ZnO sensor ( Fig. 6a,b ). The coherence function is evaluated to be unity from 100 to 800 Hz and is observed to drop below unity owing to weak piezoelectric voltage response at frequencies above 800 Hz as shown in Fig. 6c . The RMS sensitivity is calculated from 1 g amplitude sinusoidal acceleration input at frequencies ranging from 100 to 1,000 Hz and agrees well with the FRF magnitude as shown in Fig. 6d . The mean sensitivity in the ±3 dB flat region that spanned up to 350 Hz was equivalent to ~2.54 mV g −1 . V pp from the ZnO sensor is only ~3.8 mV at 200 Hz, with the maximum V pp of ~22 mV obtained at the resonant frequency of 500 Hz as shown in Fig. 6e,g with corresponding detailed shape in Fig. 6f,h , respectively (see Supplementary Fig. S10b,c for detailed shape of acceleration and voltage that is in-phase at 100 and 200 Hz, and Supplementary Fig. S10d for 90° out-of-phase relationship between acceleration and voltage near resonance at 500 Hz). The measured ±3 dB flat band sensitivity from ZnO sensor of ~2.54 mV g −1 is lower than the flat band sensitivity recorded from the novel BaTiO 3 sensor of ~50 mV g −1 , thus validating superior sensing performance of the ultra-long BaTiO 3 NW arrays as shown clearly in the magnitude comparison plot of FRF with frequency axis in a log scale ( Fig. 6i ). 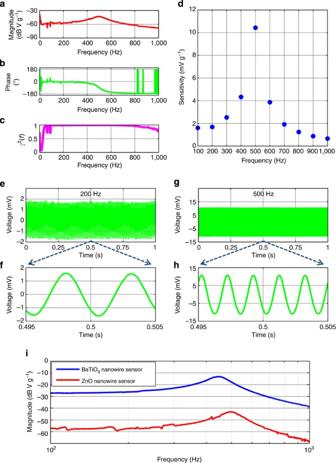Figure 6: Characterization and comparison of ZnO NW NEMS sensor. (a) FRF illustrated by magnitude in dB scale of V g−1, (b) phase angle in degree and (c) the coherence function (γ2(f)) of ZnO NW sensor obtained from white noise excitation. (d) RMS sensitivity from frequencies ranging from 100 to 1,000 Hz from sinusoidal excitation. (e) Voltage measured at 200 Hz from 1 g amplitude acceleration input with (f) showing detailed shape with aVppof ~3.8 mV. (g) Voltage measured near resonant frequency (500 Hz) showing aVppof ~22 mV from 1 g amplitude acceleration input with (h) showing the detailed shape. (i) Comparison of magnitude of the FRF with frequency axis in log scale to clearly depict the higher ±3 dB flat band sensitivity of ~50 mV g−1from BaTiO3NW sensor as compared with ±3 dB sensitivity of ~2.5 mV g−1from ZnO NW sensor. Figure 6: Characterization and comparison of ZnO NW NEMS sensor. ( a ) FRF illustrated by magnitude in dB scale of V g −1 , ( b ) phase angle in degree and ( c ) the coherence function ( γ 2 (f) ) of ZnO NW sensor obtained from white noise excitation. ( d ) RMS sensitivity from frequencies ranging from 100 to 1,000 Hz from sinusoidal excitation. ( e ) Voltage measured at 200 Hz from 1 g amplitude acceleration input with ( f ) showing detailed shape with a V pp of ~3.8 mV. ( g ) Voltage measured near resonant frequency (500 Hz) showing a V pp of ~22 mV from 1 g amplitude acceleration input with ( h ) showing the detailed shape. ( i ) Comparison of magnitude of the FRF with frequency axis in log scale to clearly depict the higher ±3 dB flat band sensitivity of ~50 mV g −1 from BaTiO 3 NW sensor as compared with ±3 dB sensitivity of ~2.5 mV g −1 from ZnO NW sensor. Full size image In summary, we have developed a novel NEMS sensor composed of ultra-long, vertically aligned BaTiO 3 NW arrays that utilizes piezoelectric behaviour to detect acceleration from mechanical vibration source. Here we simultaneously compare the NW NEMS accelerometer with a commercially available instrumentation-grade shear accelerometer to evaluate its sensing performance. This article represents the first report of the synthesis of vertically aligned BaTiO 3 NW arrays and is the first piezoelectric NW-based sensor [5] , [16] , [17] , [18] , which has been characterized to show excellent coherence, linearity and wide operating bandwidth by testing over a frequency spectrum that spans up to 10 kHz. In addition, the resonant frequency from the NW sensor can be adjusted by varying the seismic mass during the fabrication process and, thereby, provides control over the sensitivity and operating frequency bandwidth of the BaTiO 3 NW-based sensor to suit different application requirements. Furthermore, the sensitivity of BaTiO 3 NW sensor (~50 mV g −1 ) is demonstrated to be higher than the sensitivity of the ZnO NW sensor (~2.5 mV g −1 ) when direct comparison was performed under the same testing conditions. However, semiconducting ZnO NWs exhibit other useful functionalities such as the piezotronic and piezo-phototronic effects that utilize strain-induced piezo-potential as the gate voltage to tune carrier generation, transport and separation across interface/junction, which is of immense interest in nano-electronic and optoelectronic devices [36] , [37] . In conclusion, high resolution and accurate sensing of the mechanical vibration has been demonstrated using a piezoelectric sensor composed of aligned BaTiO 3 NW arrays, which can be directly grown or applied to surfaces without the clean room processing required for MEMS accelerometers. Thus, the results demonstrate new device architecture for low-cost NEMS sensors and energy harvesters. Synthesis of ultra-long, aligned BaTiO 3 NW arrays The preparation of ultra-long, aligned BaTiO 3 NW arrays involves a two-step hydrothermal reaction. First, ultra-long, vertically aligned sodium titanate NW arrays were grown on Ti substrate through a hydrothermal reaction with the Ti substrate acting as the Ti source. The Ti foil (MTI Corporation; 99.9%, 100 μm thick) was cleaned via bath sonication for 30 min in an acetone, 2-proponal and deionized water (1:1:1) solution. It was then oxidized in a furnace at 750 °C for 8 h. The resulting oxidized substrate was then immersed in a Teflon-lined autoclave filled with 37.5 ml of 12 M NaOH solution (Fill Factor: 50%, 97% Alfa Aesar) and sealed in a high-pressure reactor [38] , [39] . The reactor was placed at 210 °C in an oven for 8 h to result in the controlled growth of the sodium titanate NW arrays. After cooling the reactor, the resulting substrate was washed four times using deionized water and ethanol, and then allowed to dry at room temperature. The dried substrate with sodium titanate NW arrays is immersed in a Teflon-lined autoclave containing a barium hydroxide octahydrate (Ba(OH) 2 ·8H 2 O) solution (Fill Factor: 33%, Sigma-Aldrich), which is sealed in a reactor after filling it with argon gas. During this second hydrothermal reaction, the Ba ions diffuse into sodium titanate NWs to transform to BaTiO 3 NWs [24] . The reactor was placed in an oven at temperatures between 150 and 250 °C, and upon cooling the reactor the substrate was removed from the vessel and washed with dilute nitric acid, deionized water and ethanol. Lastly, the substrate was dried to yield the BaTiO 3 NW arrays that were used for characterization and fabrication of the NEMS sensor. Characterization of BaTiO 3 NW arrays The morphological properties, which include the orientation, dimension and crystalline structure of the as-prepared BaTiO 3 NW arrays, were examined using a JEOL 6335F SEM and an XRD equipped with a curved position-sensitive detector (CPS120, Inel) with Cu Kα radiation (see Supplementary Information for XRD pattern of all materials used in BaTiO 3 NW synthesis Supplementary Fig. S1 ). The crystal structure, lattice parameter and diffraction pattern of individual NWs were studied using the FEI Tecnai F30 (Philips) HRTEM that operates at 300 kV accelerating voltage provided by field-emission electron gun. Fabrication of NEMS BaTiO 3 NW accelerometer Borosilicate glass (1 mm thick) was used as the base substrate in the fabrication of the sensor by cutting a square (1 cm 2 ) using a laser ablator (Epilog Laser). The as-synthesized and dried film of BaTiO 3 NW arrays (6 mm × 6 mm) were removed from the oxidized Ti foil and bonded to the borosilicate glass with a uniform thin layer of conductive silver epoxy (MG Chemicals). The silver epoxy was then cured at 70 °C for 10 min to enhance the adhesion and served as the bottom electrode. A thin solder film (4 mm × 4 mm) acting as the top electrode was overlaid on top of the NW arrays and heated to 150 °C to improve the bonding with the NWs’ top surface. Signal wires were attached to the bottom and top electrode using silver epoxy. Capacitance measurement was performed using Agilent precision LCR meter (E4980A). High-voltage poling was performed by maintaining strong electric field of ~75 kV cm −1 (320 V) from a DC voltage supply (TREK, 677A Supply/Amplifier) across the signal wires of NW accelerometer for 12 h. The poling process establishes the direction of polarization along the vertical orientation of the NW arrays, and the piezoelectric coupling property in the poled axis is responsible for the voltage response from the NW accelerometer. Acceleration measurement Mechanical vibration was provided by a miniature electromagnetic shaker (Labworks, Inc., ET-132) and the voltage measurements from the sensor under vibration excitation was performed using a voltage follower/buffer amplifier with unity gain from Linear Technologies (LTC6240CS8), which was chosen for its high input resistance (1TΩ), low bias current (0.2 pA) and low noise (voltage noise <10nV/ ✓ Hz) utilized by Williams et al. [40] , [41] for AlN piezoelectric microphones. The sensor and voltage follower was placed inside a grounded faraday cage that acts as a noise shield from electromagnetic interference to improve the signal-to-noise ratio of the sensor. All signals were generated and acquired through a high-resolution (24-bit) DAQ board (NI USB 4431) operated using NI SignalExpress software. All signals were re-evaluated during data acquisition using an Oscilloscope (Tektronix, DPO 3014 Digital Phosphor Oscilloscope). Growth approach for BaTiO 3 NW arrays A hydrothermal approach is utilized here for the synthesis of aligned BaTiO 3 NW arrays, as it is of low cost, is scalable and enables control over the resulting NW morphology by tuning the reaction parameters [24] . Prior literature using the hydrothermal method for formation of BaTiO 3 nanostructures [42] , [43] clearly shows the synthesis to be highly dependent on the type of precursor, as the crystal structure and composition must accept the barium ions with a change in the precursors’ morphology. Consequently, we first hydrothermally synthesized ultra-long (~45 μm), vertically aligned single-crystal sodium titanate NW arrays on an oxidized Ti foil [38] , [39] and used them as a precursors for conversion to BaTiO 3 NW while preserving the NW form. The sodium titanate nanostructures have strong ion-exchanging properties owing to its open structure with titanium octahedra (TiO 6 ) units and was previously reported to easily convert to protonated titanate by H + /Na + ion exchange in an HCl solution [39] , [44] . The reaction parameters for the synthesis of sodium titanate NW arrays were optimized to obtain NWs with sufficient aspect ratio (~75) such that they do not wick together from the capillary forces during drying [23] . Next, these single-crystal sodium titanate NW arrays were utilized as precursors and converted to BaTiO 3 NW arrays using a second hydrothermal reaction with aqueous barium hydroxide solution in a high-pressure reactor at temperatures between 150 and 250 °C. During this second hydrothermal reaction, the Ba 2+ ions diffuse into aligned single-crystal sodium titanate NW arrays to transform into BaTiO 3 NW arrays. A step-by-step characterization was performed using the XRD to identify the material’s crystal structure, starting from the initial pure Ti foil substrate to the sodium titanate NW precursors used for synthesis of BaTiO 3 NW arrays ( Supplementary Fig. S1 ). The XRD analysis on the crystal structure of sodium titanate NW arrays used as precursors showed a majority of the peaks to match with sodium hexatitanate (Na 2 Ti 6 O 13 ) (JCPDS 31-1329) and some with sodium trititanate (Na 2 Ti 3 O 7 ) (JCPDS 73-1398) [45] , [46] . The crystal structure and lattice parameter of individual NWs were studied using HRTEM and demonstrated the transformation from single-crystal sodium titanate NW precursor to single-crystal BaTiO 3 NWs upon Ba 2+ ion exchange. Experimental characterization of BaTiO 3 NW accelerometer An accelerometer composed of the as-synthesized and dried ultra-long, aligned BaTiO 3 NW arrays was fabricated by transferring the NW arrays to a borosilicate glass substrate and using a uniform layer of silver epoxy as the bottom electrode followed by the application of a thin film of solder (Sn60Pb40) to the NW array surface, which acted as the second electrode. The sensor fabrication process is shown in Supplementary Fig. S2a,b and the cross-section of the NWs between the two electrodes with NWs adhering to the solder foil following a heating process is shown clearly in Supplementary Fig. S3a–c (see Supplementary Table S1 for the properties of the sensor). After fabrication, the capacitance ( C p ) of the NW sensor was measured to be ~2.94 pF using a high-precision LCR meter (Agilent E4980A), which validates the electrical contact made with the NWs and the absence of resistive contact between the two electrodes. The insulation resistance ( R p ) of the NW sensor is typically two orders of magnitude higher than the impedance of the source capacitance well into the GΩ range influencing the source time constant ( τ=R p *C p ). The high insulation resistance ( R p ) also reduces the low cut-off (corner) frequency limit ( f L =1/(2*π*τ) ) of the piezoelectric NW sensor. The low cut-off frequency limit contributes to the reason for the piezoelectric sensor not being able to perform true static measurements. The sensor was then poled by applying a high DC field (75 kV cm −1 ) to align the dipoles along the orientation of the NWs, which ensures that any dynamic strain applied on the NW would result in net charge generation. A poled functional sensor was then tested by inducing vibration from a miniature permanent magnet shaker, and the true input acceleration supplied to the base of the sensor is measured using a shear accelerometer (PCB352C22) that has a sensitivity of 8.81 mV g −1 . The open-circuit voltage measurements are performed using a unity gain voltage follower (LTC6240CS8) having 1 TΩ input impedance and capacitance of 3.5 pF. The cut-off frequency is lower for the voltage follower than the NW accelerometer and, hence, does not attenuate the piezoelectric voltage response at low frequencies [41] . Moreover, a voltage follower was used rather than a charge amplifier, as it offers a wider range of working frequency by not imposing a reduction in the resonant frequency because the stiffness of the piezoelectric material is at its maximum when the electrical boundary conditions are open [47] . The output voltage from the voltage follower is susceptible to the cable capacitance, which may adversely affect the sensor’s actual sensitivity, and hence the sensor is connected to the voltage follower using short low-noise cables with a grounded faraday cage surrounding the entire connection setup to reduce the noise floor ( Supplementary Fig. S4a–c ). The voltage noise floor of the sensor is estimated by the voltage spectral density acquired using NI DAQ system from the voltage follower connected to the undisturbed BaTiO 3 NW sensor ( Supplementary Fig. S6a ). By considering the true base acceleration that is measured by the reference single axis shear accelerometer (PCB 352C22) as the input to the NW sensor and the open-circuit voltage measured by the unity gain voltage follower (LTC6240CS8) as the output, the NW sensor is characterized as a NEMS-based accelerometer. Performance evaluation of the BaTiO 3 NW accelerometer The FRF and coherence function ( γ 2 (f) ) were used to evaluate the sensitivity, linearity and operating bandwidth of the NW sensor from white noise excitation that has a flat spectral density in the frequency range of 10 kHz ( Supplementary Fig. S6b ). Ten kilohertz is chosen as the test frequency range, as it was the maximum operating bandwidth of the electromagnetic shaker (Labworks, Inc., ET-132) utilized as the vibration source in the experiments. A loaded NW sensor that has an added mass on the top electrode demonstrated a resonance at 450 Hz and a high sensitivity of 50 mV g −1 in the ±3 dB flat band region that spanned up to 300 Hz under both white noise excitation as well as sine wave excitation. A comparison of the detailed shape of the input sinusoidal acceleration of 1 g amplitude and the output piezoelectric voltage generated by the NW sensor shows an in-phase relationship at 100 Hz and a 90° out-of-phase relationship at 450 Hz, which agrees well with the phase curve in the FRF observed from white noise excitation ( Supplementary Fig. S7a,b ). To confirm the presence of piezoelectricity in the ferroelectric BaTiO 3 NW arrays, the accelerometer was heated above the BaTiO 3 Curie temperature of 120 °C in a convection oven to relax the aligned dipoles to random directions and then tested to observe the loss in coherence from the reduction in piezoelectric voltage ( Fig. 5a–c ). In addition, poling/depoling/re-poling FRF analysis from the BaTiO 3 NW NEMS sensor is performed to validate that voltage response generated by the BaTiO 3 NW arrays is due to their piezoelectric behaviour ( Supplementary Fig. S8 ). Moreover, switching polarity test is performed to validate that the voltage response from the NWs is due to piezoelectric behaviour [31] , [32] . The polarity of the voltage signal ( V ) from the poled BaTiO 3 NW sensor should be the same under the same direction of mechanical deformation. Therefore, switching the polarity of the measurement instrument (voltage buffer amplifier) should cause a reversal in output signal as shown in Supplementary Fig. S9 . In addition, the influence of switchable polarization direction ( P ) on output voltage response ( V ) is investigated for BaTiO 3 NEMS sensor to substantially validate piezoelectricity from ferroelectric BaTiO 3 NW arrays ( Fig. 5d–f ) [33] . Thereby, clear demonstration of the influence of poling/depoling/re-poling and polarization direction ( P ) on the output voltage response ( V ) from the sensor composed of ferroelectric BaTiO 3 NWs is provided to conclusively substantiate piezoelectricity. Moreover, poled functional NEMS sensor composed of annealed BaTiO 3 NW arrays at 700 °C for 1 h to remove hydroxyl defects was also tested under vibration excitation, but the results recorded did not show an increase in the performance of the sensor (see Supplementary Fig. S11 ) [24] . Synthesis of aligned ZnO NW arrays To substantiate the superior sensing performance of BaTiO 3 NW arrays, a ZnO NW-based sensor was fabricated using ZnO NW arrays that were synthesized on Au-coated Si substrate (Exsil, Inc., ~500 μm thick). The Au/Si growth substrate was initially cleaned in ethanol, isopropyl alcohol and acetone (1:1:1) solution by sonication for 10 min. It was then removed and rinsed in deionized water for 2 min followed by drying at 100 °C for 5 min. The Si substrate with Au layer on top was annealed at 500 °C for 5 min to enhance crystallinity. The growth solution (Fill Factor: 40%) was prepared using 20 mM zinc nitrate hexahydrate (Zn(NO 3 ) 2 ·6H 2 O, 99%, Sigma-Aldrich) and 4% vol. ammonium hydroxide (NH 3 ·H 2 O, 28–30% wt%, Ricca Chemical Company) [34] , [35] . The Au/Si substrate was placed on top of the growth solution so that ZnO particles did not precipitate on the NW arrays. The reaction is carried out at 95 °C for 5 h in a convection oven. The resulting substrate with ZnO NW arrays on the Au surface of the Si substrate was rinsed in deionized water and dried at room temperature. This hydrothermal synthesis process was again repeated to enhance the length of ZnO NW arrays on Au/Si substrate. The microstructure of the ZnO NWs were characterized using SEM, and cross-sectional SEM image of aligned ZnO NW arrays is shown in Supplementary Fig. 10a . Fabrication and characterization of ZnO NW accelerometer The NEMS sensor using ZnO NW arrays was fabricated for direct comparison using the as-synthesized aligned ZnO NW arrays on Au/Si substrate with the similar configuration as discussed for BaTiO 3 NW-based accelerometer with the thin solder film (4 mm × 4 mm) mounted on the NW arrays as top electrode. Here the Au layer on the Si substrate on which the NW arrays were synthesized served as the bottom electrode for the ZnO NW-based NEMS sensor; hence, there was no need to transfer the NW arrays to another conductive substrate. However, sufficient insulation at the Au/Si substrate edge was needed; thus, a Dupont Kapton polyimide film was used to ensure that there was no resistive contact between the two electrodes while attaching the signal wires. The ZnO sensor was then heated to improve the bonding between the solder and ZnO NW arrays. After fabrication, the capacitance of the sensor was measured to be 4.38 pF using an Agilent LCR meter, implying that there is no resistive contact between the two electrodes. Next, the performance of the loaded ZnO NW-based accelerometer was evaluated under the same testing procedure as that used for characterizing BaTiO 3 NW sensor. How to cite this article: Koka, A. et al. High-sensitivity accelerometer composed of ultra-long, vertically aligned barium titanate nanowire arrays. Nat. Commun. 4:2682 doi: 10.1038/ncomms3682 (2013).